Monodisperse conjugated polymer particles by Suzuki–Miyaura dispersion polymerization The self-assembly of colloidal building blocks into complex and hierarchical structures offers a versatile and powerful toolbox for the creation of new photonic and optoelectronic materials. However, well-defined and monodisperse colloids of semiconducting polymers, which would form excellent building blocks for such self-assembled materials, are not readily available. Here we report the first demonstration of a Suzuki–Miyaura dispersion polymerization; this method produces highly monodisperse submicrometer particles of a variety of semiconducting polymers. Moreover, we show that these monodisperse particles readily self-assemble into photonic crystals that exhibit a pronounced photonic stopgap. Conjugated polymers constitute a promising and powerful platform for creating high-fidelity organic photonic and optoelectronic devices, such as lasers [1] , [2] , [3] , [4] , photonic bandgap materials [5] and solar cells [6] . Manufacturing such devices requires the imposition of precise nanoscopic structures within the conjugated polymer material. This is typically achieved through labor-intensive nano- and microfabrication techniques [7] , [8] , [9] . By contrast, self-assembly would offer a promising alternative, in which the spontaneous association of microscopic building blocks leads to the energy-free creation of the desired structure. To date, self-assembled three-dimensional photonic crystals of conjugated polymers have been realized in inverse configuration only; they are formed by self-assembling particles, made from passive dielectric materials such as silica or polystyrene, into colloidal crystals, backfilling the interstitial spaces with the conjugated polymer and subsequent removal of the colloidal template [5] , [10] . Ideally however, such photonic devices are prepared through self-assembly alone, without further expenditure of energy or the necessity of costly postprocessing steps. Monodisperse colloidal particles of pure conjugated polymer would be excellent building blocks for these ultimate photonic devices [11] , [12] . Although semiconducting polymer particles of polypyrrole [13] , polyaniline [14] and polythiophene [15] have been synthesized via oxidation in a dispersion polymerization, colloidal particles of light-emitting conjugated polymers have only been prepared by postpolymerization miniemulsification [16] , reprecipitation [17] or emulsion polymerization using metal-catalysed cross-coupling reactions [18] , [19] . However, these methods lead to high polydispersities [20] , inhibiting crystallization of the colloids, thus making them unsuitable for creating self-assembled periodic structures, such as photonic crystals. Direct synthetic methods to produce large quantities of monodisperse light-emitting conjugated polymer particles remain unexplored to date. In this paper, we report the direct bulk synthesis of monodisperse conjugated polymer particles by developing a novel Suzuki–Miyaura dispersion polymerization method. The flexibility of our method is highlighted by producing particles of various conjugated polymers, such as polyfluorene, poly(fluorene-alt-benzothiadiazole) and poly(thiophene-alt-benzothiadiazole). Moreover, the particle size and shape, emission spectrum and surface functionality can be accurately tuned. Owing to their monodispersity, the colloids readily self-assemble into large-scale photonic crystals, which clearly exhibit a partial photonic bandgap (stopgap). Our demonstration of Suzuki–Miyaura dispersion polymerization opens many new routes for the preparation of monodisperse particles of a wide variety of macromolecular compounds that have so far been impossible to obtain. Particles via Suzuki–Miyaura dispersion polymerization Radically initiated dispersion polymerizations are widely applied for producing monodisperse micron-sized particles of a wide variety of polymers, such as polystyrene and poly(methyl methacrylate). Dispersion polymerization of conjugated polymer particles requires the adaptation of the Suzuki–Miyaura cross-coupling reaction to this classical method, which has not yet been achieved. The reaction mixture in a dispersion polymerization is initially homogeneous, as all of the reagents, including monomer, stabilizer and polymerization initiator, are soluble in the solvent. Once the polymerization reaction is initiated, polymer chains start to grow and their solubility decreases. As soon as a critical chain length is reached, particles nucleate through phase separation of the polymer from the solvent [21] . The first hurdle in applying the homogeneous Suzuki–Miyaura polycondensation [22] , [23] to a dispersion polymerization is finding a suitable reaction medium. Low molecular weight alcohols are good solvents for conjugated monomers and simultaneously act as non-solvents for conjugated polymers; as such they form a promising medium. A requirement for the Suzuki–Miyaura reaction is the solubility of the catalyst and base, which drive the polycondensation. We use potassium tert -butoxide as the base and tetrakis(triphenylphosphine)-palladium(0) (Pd(P(Ph) 3 ) 4 ) as the catalyst. As these are not readily soluble in methanol or ethanol, we choose 1-propanol as the dispersion medium. A second requirement for a successful dispersion polymerization is the presence of a suitable stabilizer, which prevents aggregation of the particles during and after the polymerization, thus ensuring a monodisperse (polydispersity < 5%) [24] end product. We find that a copolymer of vinyl pyrrolidone and vinyl acetate ( M w ≈50 kDa) gives excellent results; moreover, the monodispersity can be improved by adding the non-ionic surfactant Triton X-45. Finally, we find that the mixing conditions are crucial for obtaining monodisperse particles; a combination of mechanical stirring and low-intensity sonication is found to give optimal results. Only mechanical stirring or overhead tumbling did not lead to monodisperse particles, whereas high-intensity sonication leads to degradation of the polymer through chain scission. The reaction is carried out at 70 °C, which is just above the T g of the conjugated polymer, consequently the surface tension between polymer and solvent ensures sphericity of the resulting colloids. Here we focus on a set of conjugated polymers with photoluminescence spectra across the entire visible spectrum. This is accomplished by using a variety of different monomers, as shown in Fig. 1a . Blue-emitting polyfluorene P1 particles are prepared by reacting dibromofluorene 1 with a diboronic acid ester fluorene 2 in a 1:1 molar ratio. Similarly, dibromofluorene 3 is coupled with 2,1,3-benzothiadiazolebisboronic acid ester 4 to obtain green-emitting particles P2 . For red-emitting colloids P4 , monomer 4 is reacted with dibromooctylthiophene 6 . Aqueous dispersions of these colloids P1 – P4 display strong photoluminescence under near ultraviolet-excitation ( Fig. 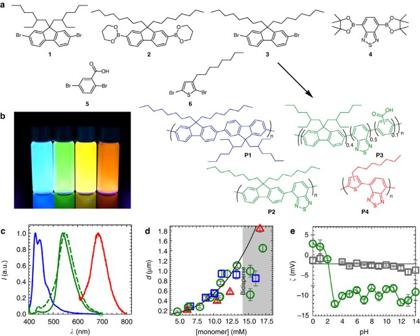Figure 1: Synthesis of monodisperse conjugated polymer particles. (a) Reaction scheme for conjugated polymer particles during a Suzuki–Miyaura dispersion polymerization with all monomers (1–6) and polymers (P1–P4) applied, (b) photograph of fluorescent dispersions of polymer particlesP1–P4in water (left to right), (c) fluorescence spectra of dispersions ofP1(blue),P2(green),P3(dashed green) andP4(red) particles, (d) particle diameterdas a function of monomer concentration forP1(blue squares),P2(green circles) andP4(red triangles). Shaded area indicates a regime where only polydisperse particles were obtained. The line is a guide to the eye. The sizes and polydispersities (s.d., represented by the error bars) were determined by SEM image analysis, except data points with thick borders; these were determined by static light scattering. (e)ζ-potential for carboxylic acid functionalizedP3particles (green circles) and unfunctionalizedP2particles (gray squares) versus the pH value of the aqueous dispersion. The lines are a guide to the eye. The error bars represent the s.d. over the number of measurements until conversion. 1b ) with quantum yields from 11–35% (see Table 1 ). This is comparable with conjugated polymer particles produced by other methods [20] , indicating that the relatively high level of palladium catalyst does not impair the optical properties of the conjugated polymer particles prepared by our new method. Clearly the fluorescence of these colloids can be tuned from blue to deep red, as shown by the corresponding spectra in Fig. 1c . The fluorescence spectra of conjugated polymer particle dispersions P1 , P2 and P4 closely resemble those of solid films of the same conjugated polymers, prepared via hetero-phase Suzuki polymerization [25] , [26] , [27] . Figure 1: Synthesis of monodisperse conjugated polymer particles. ( a ) Reaction scheme for conjugated polymer particles during a Suzuki–Miyaura dispersion polymerization with all monomers ( 1 – 6 ) and polymers ( P1 – P4 ) applied, ( b ) photograph of fluorescent dispersions of polymer particles P1 – P4 in water (left to right), ( c ) fluorescence spectra of dispersions of P1 (blue), P2 (green), P3 (dashed green) and P4 (red) particles, ( d ) particle diameter d as a function of monomer concentration for P1 (blue squares), P2 (green circles) and P4 (red triangles). Shaded area indicates a regime where only polydisperse particles were obtained. The line is a guide to the eye. The sizes and polydispersities (s.d., represented by the error bars) were determined by SEM image analysis, except data points with thick borders; these were determined by static light scattering. ( e ) ζ -potential for carboxylic acid functionalized P3 particles (green circles) and unfunctionalized P2 particles (gray squares) versus the pH value of the aqueous dispersion. The lines are a guide to the eye. The error bars represent the s.d. over the number of measurements until conversion. Full size image Table 1 Parameters for particles prepared via Suzuki–Miyaura dispersion polymerization. Full size table Monodisperse conjugated polymer particles The Suzuki–Miyaura dispersion polymerization of P2 yields monodisperse particles with a typical polydispersity of <4%, as ascertained by static light scattering (see Supplementary Fig. S2a,b ). (Analysis via scanning electron microscopy (SEM) image analysis is less accurate and gives an upper limit for polydispersity of 10%, see Supplementary Fig. S2c–j ). The size of the P2 particles can be tuned between 150 nm and 1.1 μm by changing the total concentration of monomer between 5 and 14 mM, while maintaining polydispersities <4%, as shown in Fig. 1d , Supplementary Table S1 and Supplementary Fig. S2 . Higher concentrations of monomer lead to bidispersity (see Fig. 2d ) or polydispersity in the final product, as summarized in Fig. 1d . Excellent monodispersity is supported by the fact that the particles readily crystallize upon drying ( Fig. 2a,b ). Such high monodispersities have so far not been achieved in light-emitting polymer particles regardless of the method of preparation. The monodispersity we report here is similar to that for particles of poly(methyl methacrylate) or polystyrene, prepared by using a dispersion polymerization procedure [21] . A close up of the particles reveals that the surface is smooth and does not show any roughness on scales larger than 10 nm ( Fig. 2c ). Also for the polymers P1 and P4 (see Fig. 2e,f ) monodisperse particles of tunable size can be obtained in the same range of monomer concentrations ( Fig. 1d and Supplementary Figs S1 and S3 ), thus highlighting the versatility of our method. The total conversion of these dispersion polymerizations is consistently around 55%, and moderate molecular weights for P1 , P2 and P4 are found between 13 and 17.5 kDa with polydispersities ( M n / M w ) of the polymers between 2.5 and 5 (see Table 1 ). These values for conversion and molecular weight are among the highest reported for conjugated polymer particles, prepared by a direct synthetic procedure [20] . 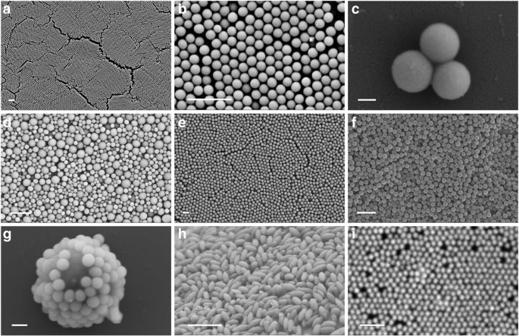Figure 2: Conjugated polymer particle assemblies. Scanning electron micrographs: (a) Crystalline sample of 420 nm sized monodisperse particles ofP2, (b) close up of 420 nmP2particles, (c) extreme close up of three 420 nmP2particles, (d) bidisperse particles ofP2, (e) 915 nm sized monodisperse particles ofP1, (f) 517 nm sized monodisperse particles ofP4, (g) a conjugated polymer particleP3covered with aminated-silica particles attached via EDC–NHS coupling to the carboxylic acid moiety ofP3, (h) ellipsoidal particles of stretched monodisperseP2particles, (i) confocal-microscopy image of crystalline 310 nm particles ofP2.(Scale bars are 2 μm except for (c) and (g) where the scale bars represent 200 nm). Figure 2: Conjugated polymer particle assemblies. Scanning electron micrographs: ( a ) Crystalline sample of 420 nm sized monodisperse particles of P2 , ( b ) close up of 420 nm P2 particles, ( c ) extreme close up of three 420 nm P2 particles, ( d ) bidisperse particles of P2 , ( e ) 915 nm sized monodisperse particles of P1 , ( f ) 517 nm sized monodisperse particles of P4 , ( g ) a conjugated polymer particle P3 covered with aminated-silica particles attached via EDC–NHS coupling to the carboxylic acid moiety of P3 , ( h ) ellipsoidal particles of stretched monodisperse P2 particles, ( i ) confocal-microscopy image of crystalline 310 nm particles of P2 . (Scale bars are 2 μm except for ( c ) and ( g ) where the scale bars represent 200 nm). Full size image Anisotropic conjugated polymer particles The spherical particles can be used to form simple self-assembled nano-structures, but the possibilities can be greatly expanded by introducing anisotropy or anisometry in the building blocks and their interactions [28] . For example, anisometric particles could allow the fabrication of crystals with controlled geometric degeneracy of the photonic bandgap [29] . We fabricate ellipsoidal particles of our conjugated polymer colloids using an established method [30] . Dry films of poly(vinyl alcohol) (PVA), containing dispersed conjugated polymer particles, are heated to above the T g of the conjugated polymer and are subsequently stretched. The particles are recovered by dissolution of the PVA matrix. Prolate ellipsoids of conjugated polymer particles that are highly monodisperse in both size and shape are obtained, as shown in Fig. 2h . These monodisperse conjugated polymer particles, both spherical or anisometric, could be excellently suited for fluorescent tagging or as tracers in biological experiments, such as flow cytometry [31] or in vivo microrheology [32] . Conjugated polymers exhibit high optical gain and excellent photostability compared with most organic dyes, although being of low cytotoxicity, thus enabling its use in living organisms without disturbing biological function [33] . Indeed, excitation with a wavelength of 488 nm, commonly available on commercial confocal or fluorescence microscopes, allows the green particles to be easily observed, as shown in Fig. 2i . A prerequisite for their use in biological experiments is that the surface of the particles can be easily modified, to allow the covalent attachment of proteins, antibodies or other molecules. To accomplish this, we prepare conjugated polymer particles with carboxylic acid moieties on the surface, such that a wide variety of molecules can be coupled for example through amide coupling, facilitated by 1-ethyl-3-(3-dimethylaminopropyl)carbodiimide and N -hydroxysuccinimide (EDC–NHS) [34] . Monomers 1 , 4 and dibromobenzoic acid 5 are polymerized in a 4:5:1 ratio, respectively ( Fig. 1a ). For this ternary copolymer, the different reactivities of the three monomers result in polymer chains of disparate composition and solubility; consequently, polymer chains precipitate at different molecular weights and particle nuclei of different sizes form. Therefore, the polydispersity of the final product P3 is significantly larger than that for the binary copolymers (>10%). To verify the incorporation of the carboxylic acid groups and their localization at the particle surface, we measure the ζ -potential of the P3 particles as a function of pH. We indeed find that the particles adopt a negative charge at pH >2.5 ( Fig. 1e ), which corresponds to the p K a of benzoic acid in a π-conjugated system [35] . Note that the particles become weakly cationic under very acidic conditions, which is possibly due to protonation of the stabilizer. As expected, particles made from the green-emitting polymer without the benzoic acid moieties carry no significant charge over the entire range of pH values explored here (gray squares in Fig. 1e ). To further confirm that the carboxylic acid moieties are accessible, we perform a standard EDC–NHS coupling of an aminosilane to the conjugated polymer particles, giving a trimethoxy-silane functionalized surface. Subsequently, 160-nm silica particles are then attached to the silane groups on the surface, resulting in a core–shell morphology of a monolayer of silica nanoparticles on the P3 conjugated polymer core particle ( Fig. 2g ). Interestingly, even small amounts (10 mol%) of the benzoic acid in the backbone of the conjugated polymer cause a red shift in the fluorescence emission ( Fig. 1b,c ). One of the most promising applications of these conjugated polymer particles is their self-assembly into semiconducting colloidal crystals, which exhibit a partial or full photonic bandgap. Light, or electromagnetic waves, with frequencies within this bandgap get reflected or entrapped inside the photonic crystal. These materials could for example be used as wavelength-specific filters, mirrors or as resonators for polymer photonics. To prepare the particles for self-assembly, they are cleaned to remove excess stabilizer and dispersed either in water containing sodium dodecyl benzene sulphonate (SDBS) or in 1-propanol with dioctyl sodium sulfosuccinate to provide electrostatic stabilization of the colloids. The particle suspensions are stable and the colloids do not aggregate over time, which was confirmed by dynamic light scattering measurements over the course of 3 days. Large crystalline arrays can be prepared by slowly drying a suspension of these particles on a precleaned glass slide. An example of such a crystal of P2 particles with a diameter of 310 nm can be seen in Fig. 3a . 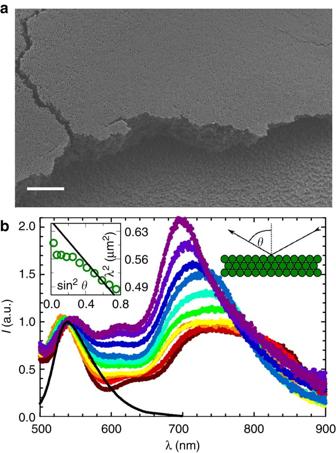Figure 3: Optical performance of a conjugated polymer colloidal crystal. (a) SEM image of a large colloidal crystal consisting of multiple crystalline domains. (b) Photoluminescence and reflectance spectra of an fcc colloidal crystal of 310 nmP2particles (symbols) at different reflection angles fromθ=60°–10° (top to bottom), all curves are normalized to the photoluminescence maximum. The corresponding photoluminescence spectrum is shown as a solid line. The insets show the square of the peak position as a function of the squared sine of the reflection angle, comparing experimental data (circles) to the theoretical prediction (solid line) and a schematic of the measurement setup, indicating the angle of reflectionθ. (Scale bar is 10 μm). Figure 3: Optical performance of a conjugated polymer colloidal crystal. ( a ) SEM image of a large colloidal crystal consisting of multiple crystalline domains. ( b ) Photoluminescence and reflectance spectra of an fcc colloidal crystal of 310 nm P2 particles (symbols) at different reflection angles from θ =60°–10° (top to bottom), all curves are normalized to the photoluminescence maximum. The corresponding photoluminescence spectrum is shown as a solid line. The insets show the square of the peak position as a function of the squared sine of the reflection angle, comparing experimental data (circles) to the theoretical prediction (solid line) and a schematic of the measurement setup, indicating the angle of reflection θ . (Scale bar is 10 μm). Full size image To verify that this crystal exhibits a partial photonic bandgap, we measure the spectrally resolved reflection of white light, incident to the (111) plane of the polycrystalline face-centered cubic (fcc) colloidal crystal. We clearly observe a partial photonic bandgap at wavelengths of approximately 700 nm, as shown in Fig. 3b . The reflection peak shifts to longer wavelengths with decreasing angle (circles in inset of Fig. 3b ); this is in good agreement with the theoretical trend (solid line) calculated with Bragg′s law for reflection from the fcc (111) plane: where d is the particle diameter, n =1.7, the refractive index of the polymer [36] and θ the angle of reflection. We attribute the sharpening of the reflectance peak with increasing angle to the systematic change in refractive index ratio between particles and interstitial spaces in other fcc planes, for example (200),(220) and (311) [37] . In addition, the reflectance spectra show green fluorescence at 550 nm, corresponding to the fluorescence of dry P2 particles, excited at 470 nm (solid line in Fig. 3b ). The reflectance spectra are normalized to the fluorescence peak, to gain a measure of the reflection intensity. This is possible due to the omnidirectional nature of the photoluminescence, its linear dependence to the excitation density and due to the fact that for this sample the emission does not overlap with the stopgap of the structure. In summary we report the first application of a Suzuki–Miyaura dispersion polymerization, resulting in highly monodisperse conjugated polymer particles. Their size, emission characteristics, surface functionality and shape can be accurately controlled by adjusting the synthetic protocol. These colloids readily self-assemble into photonic crystals that exhibit a clear photonic bangap, highlighting their potential as novel building blocks for self-assembled photonic materials. Such materials will be interesting for various applications in photonics, for example for telecommunications or optical sensing, as the conjugated polymer photonic crystal acts as both a filter and a frequency converter via photoluminescence. It absorbs in the blue and ultraviolet spectrum, emits green light and has a partial bandgap in the red part of the spectrum. The novel Suzuki–Miyaura dispersion polymerization can be applied to a wide variety of monomers opening up synthetic pathways to produce monodisperse colloidal particles and novel materials, which have so far been impossible to obtain. Synthetic procedures for conjugated polymer particles All materials were purchased from Sigma-Aldrich and used without further purification. Mixing of the reaction was accomplished using mechanical stirring and ultrasonication. A Sonics & Materials Inc GEX 600-5 tip sonicator was used. The procedure is described in detail for Poly(dioctylfluorene-alt-diethylhexylfluorene) ( P1 ), the other particles were prepared in the same manner. For particles P1 , a 20-ml glass vial was charged with equal molar amounts of 9,9-bis(2-ethylhexyl)-2,7-dibromofluorene 1 and 9,9-dioctylfluorene-2,7-diboronic acid bis(1,3-propanediol)ester 2 (see Supplementary Table S1 for amounts of individual batches), 720 mg of poly(1-vinylpyrrolidone-co-vinyl acetate) (avg. MW=50,000 Da, ~1.3:1 mole ratio of VP:VA), 800 mg of Triton X-45 and 6.6 ml of 1-propanol. After these materials had dissolved, the mixture was filtered (0.45 μm, polytetrafluoroethylene (PTFE) syringe filter) into a precleaned 25 ml flask. After degassing for at least 10 min by bubbling with argon, 1 mg tetrakis(triphenylphosphine)-palladium(0) catalyst was added. The reaction flask was then charged with a stirrer bar and sealed with a rubber septum, and degassed with argon for another 10 min. The nozzle of the tip-sonicator was inserted through an opening in the septum until the tip was ca. 2 mm beneath the surface of the reaction mixture. The flask was transferred into a 70 °C oil bath and stirred magnetically (1,300 r.p.m. ), while the tip-sonicator was operated continuously at 12 W. After 5 min, when all of the the catalyst had dissolved, 1.4 ml of a degassed solution of 5 g l −1 potassium tert -butoxide in 1-propanol was added to initiate the polymerization. The reaction mixtures turned turbid within 30 min and the reaction was left to react to completion between 30 min and 4 h. Yield after purification: 56%, 1 H-NMR (500 MHz, CDCl 3 ) δ (ppm): 7.90–7.80 (broad, 2H, ArH), 7.75–7.55 (broad, 4H, ArH), 1.26-1.05 (broad, 11H, CH 2 , CH), 1.02–0.75 (broad, 14H, CH 2 ), 0.70–0.55 (m, 9H, CH 3 ). Amount of incorporated poly(1-vinylpyrrolidone-co-vinyl acetate) (PVPVA) is between 5 wt% (determined by 1 NMR) and 7 wt% (determined by elemental analysis). Anal. calculated for C 29 H 40 with 7 wt% stabilizer: C: 83.63, H: 9.63, N: 0.71; found: C: 82.99, H: 9.699, N: 3.17, S: 0.882. Poly(dioctylfluorene-alt-benzothiadiazole) ( P2 ) particles: equal molar amounts of 2,1,3-benzothia-diazole-4,7-bis(boronic acid pinacol ester) 4 and 9,9-dioctyl-2,7-dibromofluorene 3 (see Fig. 1d and Supplementary Table S1 ) were applied with 2 mg Pd((PPh 3 ) 4 ): Yield after purification: 54%, 1 H-NMR (500 MHz, CDCl 3 ) δ (ppm): 8.10–7.90 (broad, 3H, ArH), 7.90–7.50 (dd, 1H, ArH), 1.24–1.05 (broad, 12H, CH 2 ), 1.03–0.90 (broad, 2H, CH 2 ), 0.86–0.72 (m, 3H, CH 3 ). Amount of incorporated PVPVA is between 8 wt% (determined by 1 NMR) and 7.5 wt% (determined by elemental analysis). Anal. calculated for C 35 H 42 N 2 S with 7.5 wt% stabilizer: C: 74.40, H: 7.40, N: 6.07, S: 5.67 found: C: 74.99, H: 7.729, N: 6.09, S: 5.31. Poly(diethylhexyl-co-benzothiadiazole- co -benzoic acid) ( P3 ) particles were obtained when using 22.5 mg 9,9-bis(2-ethylhexyl)-2,7-dibromofluorene 1 (0.041 mmol), 21.0 mg 2,1,3-benzothiadiazole-4,7-bis(boronic acid pinacol ester) 4 (0.054 mmol) and 3.7 mg 2,5-dibromobenzoic acid 5 (0.013 mmol) with 2 mg of tetrakis-(triphenylphosphine)-palladium(0) catalyst. Polydisperse particles with a mean size around 700 nm were obtained at a yield of 16.8 mg after purification (55%), 1 H-NMR (500 MHz, CDCl 3 ) δ (ppm): 8.50–8.58 (broad, 0.1H, OH), 8.18–7.90 (broad, 3H, ArH), 7.90–7.60 (dd, 1H, ArH), 7.48–7.52 (m, 0.3H, ArH), 1.24–1.06 (broad, 7H, CH 2 , CH), 1.00–0.86 (broad, 4H, CH 2 ), 0.88–0.73 (m, 6H, CH 3 ). Amount of incorporated PVPVA 22 wt% (determined by 1 NMR). Poly(thiophene-alt-benzothiadiazole) ( P4 ) particles: equal molar amounts of 2,1,3-benzothiadiazole-4,7-bis(boronic acid pinacol ester) 4 and 2,5-dibromo-3-octylthiophene 6 (see Fig. 1d and Supplementary Table S1 ) were applied with 1.5 mg Pd((PPh 3 ) 4 ): Yield after purification: 56%, 1 H-NMR (500 MHz, CDCl 3 ) δ (ppm): 8.30–7.70 (broad, 3H, ArH), 2.88–2.72 (broad, 2H, CH 2 ), 1.44–1.10 (broad, 10H, CH 2 ), 0.80–0.94 (m, 3H, CH 3 ). Amount of incorporated PVPVA 12 wt% (determined by 1 NMR). See Supplementary Table S1 in the Supplementary Information for monomer amounts and particle yields of all other P1 , P2 , P4 particles studied in this study. Purification. The particles were separated from the reaction mixture by centrifugation and resuspended in a 0.5 wt% solution of SDBS or dioctyl sodium sulfosuccinate in 1-propanol or 5 wt% of SDBS in water; this is repeated at least five times. The particles are then washed two more times with pure 1-propanol or DI water, before SEM analysis or further experiments. All characterization experiments were performed on cleaned particles. (Except for ζ -potential measurements, particles were only washed with water). Ellipsoidal conjugated polymer particles. 0.1 wt% of P2 (420 nm) particles were added to a 10 wt% solution of PVA (avg. M w =205,000 Da) in water with 5% glycerol (to PVA). This mixture was poured into petri dishes and left to dry for 48 h to create dry composite films. The rectangular section of one of these films was clamped into a home-build stretching device, which was immersed into a 150 °C oil bath and heated for 10 s, after which the film was stretched over a period of 10 s. The film was then cooled and excess mineral oil was removed by soaking the film in 1-butanol for 30 min. The film was subsequently immersed in water to dissolve the PVA matrix. The colloids were obtained and purified by several centrifugation and washing cycles. The particles were redispersed to produce a ~50 wt% dispersion in 1-propanol for SEM analysis. Coupling of silica particles to carboxylated conjugated polymer particles. P3 particles were washed by centrifugation and redispersion with water for at least 10 times. The particles were then dispersed in a 100 mM solution of 4-(2-hydroxyethyl)-1-piperazineethanesulfonic acid buffer (pH=8) and EDC–NHS and 3-aminopropyltriethoxy silane were added in excess. The dispersion was tumbled for 12 h. The excess reagents were separated from the particles by centrifugation and redispersion of the particles in water. Then an excess of 160 nm silica particles, suspended in a solution of 0.1 M ammonium hydroxide, was added. The dispersion was tumbled for 6 h and then purified to remove excess silica particles. The particles were redispersed in water for SEM analysis. Reflectance measurements. Reflectance measurements were performed by coupling an optical fiber to a broad spectrum white light source. A collection fiber was coupled to a spectrometer. Both fibers were fitted to a goniometer. The illumination and collection fibers were aligned on the photonic crystal and the reflection spectra from angles between 10° and 60° were recorded. Polymer molecular weights. Molecular weights were determined by gel permeation chromatography using a Waters/Millipore UV detector 481 and a size exclusion column combination (Latek Styragel 50/1,000 nm pore size). All gel permeation chromatography measurements were carried out using freshly distilled tetrahydrofuran at 45 °C. The columns were calibrated versus commercially available polystyrene standards. Confocal microscopy. Confocal microscopy images were recorded on a Leica SP5 confocal microscope, equipped with a X100 (1.4 NA) immersion objective and excitation at 488 nm. Scanning electron microscopy. The particles were deposited from their dispersions by drying in air. After drying the colloidal assemblies were sputter coated with a 5–10 nm film of gold before SEM analysis. The images were recorded on a Zeiss Supra SEM at 5 kV using Everhart–Thornly and Inlens detectors. Particle size and characterization. Particle sizes were determined from SEM images of crystalline as well as submonolayer colloidal samples (as indicated in Supplementary Table S1 ) of P1 , P2 and P4 . ImageJ analysis software was used to determine the particle size distribution from the SEM images. Alternatively, P1 and P2 particles were sized using static- and dynamic light scattering, while the data were analysed using MiePlot ( http://www.philiplaven.com ) and AfterALV ( http://www.dullware.nl ), respectively. The distributions obtained from image analysis were fitted with a Gaussian/normal distribution giving the mean sizes and s.d., as presented in Fig. 1d and Supplementary Figs S1–S3 . The static light scattering data were fitted with a classic BHMIE (Bohren, Huffman, Mie-) scattering algorithm assuming a log-normal distribution. From this distribution the particle mean sizes and s.d. were extracted, which are presented in Fig. 1d as thick symbols and in Supplementary Figs S1a and S2a,b . The polydispersity expressed in percent is calculated by dividing the s.d. by the peak mean in the particle size distribution. ζ -potential measurements. The ζ -potentials of dilute aqueous dispersions of P2 and P3 were measured on a Malvern Instruments Zetasizer Nano. Samples from pH=0–14 were measured. Each sample was checked until conversion occurred. Data-points for sample P2 at pH=2 and 3 were excluded as no consistent values were found after 100 measurements. Particle photoluminescence. Fluorescence spectra of dilute aqueous dispersions of P1 – P4 were recorded on a custom build fluorescence spectrometer. P1 – P3 were excited at 380 nm and P4 was excited at 580 nm. Photoluminescence Quantum Yields of butanol dispersions of all types of particles P1 – P4 were determined on a Hamamatsu Ulbricht-sphere. P1 – P3 were excited at 380 nm and P4 was excited at 630 nm. How to cite this article: Kuehne, A.J.C. et al . Monodisperse conjugated polymer particles by suzuki–miyaura dispersion polymerization. Nat. Commun. 3:1088 doi: 10.1038/ncomms2085 (2012).